Thrombin-dependent intravascular leukocyte trafficking regulated by fibrin and the platelet receptors GPIb and PAR4 Thrombin is a central regulator of leukocyte recruitment and inflammation at sites of vascular injury, a function thought to involve primarily endothelial PAR cleavage. Here we demonstrate the existence of a distinct leukocyte-trafficking mechanism regulated by components of the haemostatic system, including platelet PAR4, GPIbα and fibrin. Utilizing a mouse endothelial injury model we show that thrombin cleavage of platelet PAR4 promotes leukocyte recruitment to sites of vascular injury. This process is negatively regulated by GPIbα, as seen in mice with abrogated thrombin-platelet GPIbα binding ( hGPIb α D277N ). In addition, we demonstrate that fibrin limits leukocyte trafficking by forming a physical barrier to intravascular leukocyte migration. These studies demonstrate a distinct ‘checkpoint’ mechanism of leukocyte trafficking involving balanced thrombin interactions with PAR4, GPIbα and fibrin. Dysregulation of this checkpoint mechanism is likely to contribute to the development of thromboinflammatory disorders. The protease α-thrombin plays a central role in linking blood coagulation with platelet activation and inflammation [1] , [2] , [3] . Thrombin has pleiotropic effects within the vasculature, principally through the generation of fibrin and via the stimulation of cells through cleavage of protease-activated receptors (PARs). PARs are found on the surface of many cell types including platelets, endothelial cells, smooth muscle cells as well as effector cells of the immune system [4] , [5] . Thrombin activation of platelets through PARs is central to their haemostatic and prothrombotic functions [6] , [7] and leads to the generation and release of a broad range of proinflammatory molecules [8] , [9] . Thrombin activation of endothelial and immune effector cells induces the production of several growth factors, chemokines and cytokines [4] , [10] , [11] and also alters their adhesive phenotype [12] , [13] . Thrombin stimulation of endothelial cells via PAR1 induces signalling predominantly via the NF-κB pathway, resulting in the expression of a broad range of chemokines including interleukin (IL)-6 (ref. 14 ), IL-8 (ref. 14 ), platelet activating factor (PAF) (ref. 15 ) and monocyte chemoattractant protein-1 (MCP-1) (ref. 11 ), proangiogenic mediators such as transforming growth factor-β (ref. 3 ) and pro-adhesive molecules including intercellular adhesion molecule-1 (ICAM-1) (refs 12 , 13 ) and P-selectin [12] that act cooperatively to enhance leukocyte recruitment and inflammation [3] . However, the relative importance of these thrombin-initiated signalling events in endothelial cells, relative to the activation of platelets, in promoting efficient recruitment and trafficking of leukocytes to sites of endothelial perturbation remains poorly defined. In addition to its catalytic activity, thrombin’s biological function is critically dependent on its binding interactions with a broad range of target proteins [16] , [17] . Foremost among these are fibrin and platelet GPIbα, the two major thrombin-binding partners within a developing thrombus. Thrombin has two basic anion-binding exosites (exosite I and II) that bind to all natural cofactors and substrates of thrombin. Exosite I binds fibrin, hirudin [18] , Heparin Cofactor II, PARs, thrombomodulin and various coagulation factors [16] , [19] . Exosite II is the major heparin-binding site [20] , but can also interact with highly sulfated polysaccharides and γ′-fibrinogen [21] . These exosites are also important for α-thrombin binding to GPIbα, the principal thrombin-binding site on platelets [22] , [23] , [24] . The importance of the GPIbα/exosite I and II interaction in promoting thrombin binding to GPIbα has been well defined [22] , [25] , [26] . However, despite more than 30 years of investigation and two published crystal structures [23] , [24] , the precise pathophysiological function of the thrombin–GPIbα interaction remains unclear. Progress in defining the molecular mechanisms by which thrombin promotes leukocyte recruitment to sites of endothelial perturbation in vivo has been hampered by a paucity of well-controlled animal models of localized leukocyte recruitment linked to the activation of blood coagulation. For example, while laser injury to the microvasculature [27] , [28] or the topical application of ferric chloride in the mouse microcirculation [29] leads to the activation of coagulation, thrombin generation and platelet thrombus formation, these models do not typically induce robust leukocyte recruitment and trafficking responses at the injured vessel wall. Part of this may be related to the study of thrombosis in the arterial circulation, where leukocyte–vessel wall interactions are far less prominent than in venules or veins. We have therefore developed a microvascular traumatic needle injury model that results in localized endothelial injury in the mesenteric venous circulation, leading to thrombin generation, fibrin accumulation and a highly reproducible platelet and leukocyte recruitment response [30] . A key feature of this model is the ability to microinject pharmacological agents precisely at sites of platelet and leukocyte accumulation on the injured endothelium, which when combined with genetically manipulated mouse models, represents a potentially powerful approach to dissect the molecular pathways regulating intravascular leukocyte recruitment and trafficking. Utilizing this model, we find that the predominant mechanism by which thrombin promotes leukocyte recruitment to the injured vessel wall is through the activation of platelets, not endothelial cells, via platelet PAR4. Notably, firm leukocyte adhesion and intravascular migration through platelet thrombi occur independent of fibrin generation. Indeed, fibrin appears to play an important role in limiting leukocyte recruitment and migration at least partially through the sequestration of α-thrombin, and also by acting as a physical barrier to the migration of leukocytes through platelet thrombi. Likewise, disrupting thrombin binding to GPIbα enhances platelet activation and leukocyte recruitment, suggesting that GPIbα may have a negative effect on thrombin’s proinflammatory function. Overall, these studies define a distinct regulatory mechanism controlling the trafficking of leukocytes to sites of vascular injury that is dependent on multiple catalytic and substrate-binding functions of thrombin. Procoagulant endothelial cells recruit platelets and leukocytes To gain insight into the mechanisms by which α-thrombin promotes leukocyte recruitment to sites of vascular injury, we utilized a traumatic needle injury model of endothelial perturbation in the mesenteric venous circulation of mice [30] . In this model, injury to the endothelium was associated with phosphatidylserine (PS) exposure on the cell surface ( Fig. 1a and Supplementary Fig. 1 ), which increased rapidly over the first 5 min following injury ( Supplementary Fig. 1 ). Endothelial PS exposure supports the assembly of coagulation complexes on the cell surface, leading to thrombin generation [31] , [32] . Consistent with this, staining of the endothelium with an anti-fibrin monoclonal antibody revealed localized fibrin generation at the sites of needle injury, confirming α-thrombin generation ( Fig. 1b ). The PS-positive (PS+ve) endothelial cells were highly reactive to platelets such that following needle injury, platelet thrombus formation occurred exclusively on PS+ve endothelial cells ( Fig. 1c ). These regions of platelet accumulation on the PS+ve endothelium were highly efficient at recruiting leukocytes and inducing leukocyte migration ( Fig. 1d ). Systemically infusing mice with the direct thrombin inhibitor, hirudin (50 mg kg −1 ), inhibited stable platelet thrombus formation and eliminated leukocyte recruitment and intravascular migration ( Fig. 1e–g ). Furthermore, localized microinjection of thrombin at the site of needle injury markedly increased the number of leukocytes that developed a polarized morphology and subsequently underwent directed migration towards the initial site of injury ( Fig. 1f,g ), indicating a central role for α-thrombin in regulating leukocyte recruitment and trafficking to sites of endothelial injury in this model. 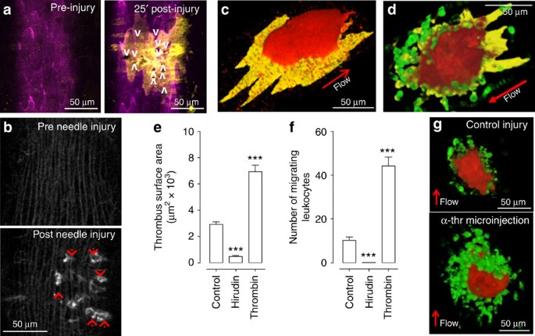Figure 1: Thrombin regulation of leukocyte recruitment at sites of vascular injury. C57BL/6J mice were systemically administered Alexa 488-Annexin V, Alexa 488-anti-fibrin Ab, DyLight 649 anti-GPIbβ Ab and PE-Gr-1 Ab, where indicated, to monitor PS exposure, fibrin generation, and platelet and leukocyte adhesion, respectively. In some experiments, mice were administered hirudin (50 mg kg−1) before injury. Mesenteric needle injury was induced as detailed under ‘Methods’ and the mesenteric vasculature subjected to DIC and confocal intravital microscopy. (a) Representative fluorescence images demonstrating PS positivity (yellow) pre- and 25 min post injury (PS: yellow; anti-PECAM Ab: magenta; note: each arrow head (V) represents a site of initial endothelial injury). (b) Representative DIC/fluorescence images demonstrating fibrin formation (white) pre- and post-injury (note: each arrow head (V) represents a site of initial endothelial injury.). (c) Representative images demonstrating platelet thrombi (red) formed on the PS+ve endothelial surface (yellow) post injury. (d) Representative image demonstrating adherent as well as polarized/migrating leukocytes (green) within the body of a platelet thrombus (red) on PS+ve endothelium (yellow) post injury. (e–g) Thrombotic responses and leukocyte–thrombus interactions were examined in vehicle (Control) and hirudin-administered mice, in the absence or presence of local microinjection of thrombin (Thrombin). Thrombus surface area (e) and leukocyte migration (f) were quantified 20 min post injury, as described in ‘Methods’. Results represent the mean±s.e.m. (n=35 injuries (control);n=31 injuries (thrombin);n=10 injuries (hirudin)), where***P<0.001.Pvalue was calculated by one-way analysis of variance (ANOVA) with Dunnett’s post testing. (g) Representative three-dimensional (3D) reconstructed confocal images depicting leukocyte recruitment (green) and platelet thrombi (red) in the absence (control injury) or presence of microinjected thrombin (α-thr microinjection). Scale bar, 50 μm. Figure 1: Thrombin regulation of leukocyte recruitment at sites of vascular injury. C57BL/6J mice were systemically administered Alexa 488-Annexin V, Alexa 488-anti-fibrin Ab, DyLight 649 anti-GPIbβ Ab and PE-Gr-1 Ab, where indicated, to monitor PS exposure, fibrin generation, and platelet and leukocyte adhesion, respectively. In some experiments, mice were administered hirudin (50 mg kg −1 ) before injury. Mesenteric needle injury was induced as detailed under ‘Methods’ and the mesenteric vasculature subjected to DIC and confocal intravital microscopy. ( a ) Representative fluorescence images demonstrating PS positivity (yellow) pre- and 25 min post injury (PS: yellow; anti-PECAM Ab: magenta; note: each arrow head (V) represents a site of initial endothelial injury). ( b ) Representative DIC/fluorescence images demonstrating fibrin formation (white) pre- and post-injury (note: each arrow head (V) represents a site of initial endothelial injury.). ( c ) Representative images demonstrating platelet thrombi (red) formed on the PS+ve endothelial surface (yellow) post injury. ( d ) Representative image demonstrating adherent as well as polarized/migrating leukocytes (green) within the body of a platelet thrombus (red) on PS+ve endothelium (yellow) post injury. ( e – g ) Thrombotic responses and leukocyte–thrombus interactions were examined in vehicle (Control) and hirudin-administered mice, in the absence or presence of local microinjection of thrombin (Thrombin). Thrombus surface area ( e ) and leukocyte migration ( f ) were quantified 20 min post injury, as described in ‘Methods’. Results represent the mean±s.e.m. ( n =35 injuries (control); n =31 injuries (thrombin); n =10 injuries (hirudin)), where *** P <0.001. P value was calculated by one-way analysis of variance (ANOVA) with Dunnett’s post testing. ( g ) Representative three-dimensional (3D) reconstructed confocal images depicting leukocyte recruitment (green) and platelet thrombi (red) in the absence (control injury) or presence of microinjected thrombin (α-thr microinjection). Scale bar, 50 μm. Full size image Thrombin-activated platelets promote leukocyte trafficking Thrombin has multiple effects in the vasculature [4] , foremost among these are platelet stimulation and fibrin generation. To investigate whether the primary effect of thrombin on leukocyte migration was related to platelet stimulation, we performed studies on PAR4 −/− mice, as platelets from these mice are completely unresponsive to thrombin stimulation [33] . Compatible with a reduction in thrombin-induced platelet activation, thrombus stability in mesenteric veins was markedly decreased in PAR4 −/− mice following needle injury ( Fig. 2a,b ). Furthermore, PAR4 −/− mice had a major defect in leukocyte recruitment and migration ( Fig. 2c ), suggesting that thrombin-stimulated platelets are important for the leukocyte recruitment and trafficking response. To investigate this further we activated PAR −/− platelets in vivo by microinjecting the platelet agonist collagen-related peptide (CRP) and ADP at sites of vascular injury. This led to the formation of stable platelet thrombi and rescued the leukocyte recruitment and migratory response ( Fig. 2a,c ). Taken together, these results suggest that potent platelet stimulation is important for leukocyte recruitment and migration at sites of endothelial injury. 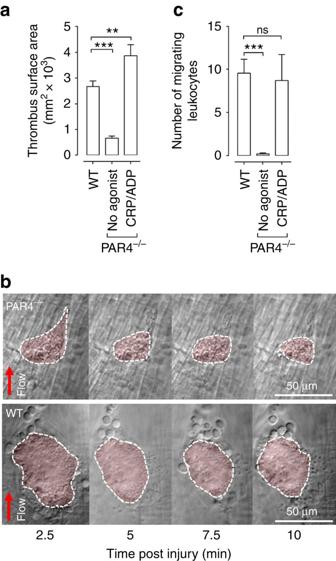Figure 2: Thrombin activation of platelets promotes leukocyte recruitmentin vivo. C57BL/6J (WT) orPAR4−/−mice were systemically administered DyLight 649 anti-GPIbβ Ab and PE-Gr-1 Ab before needle injury of mesenteric veins. (a) Thrombus surface area was quantified in the absence (no agonist) or presence of locally microinjected CRP and ADP (CRP/ADP), 20 min post injury as described in ‘Methods’. (b) Representative DIC images demonstrating thrombus instability in PAR4/mice as compared with C57BL/6J mice (WT) at the indicated times post injury (thrombus shaded in pink). (c) Leukocyte migration was quantified in the absence (no agonist) or presence of locally microinjected CRP and ADP (CRP/ADP), 20 min post injury as described in ‘Methods’. Results represent the mean±s.e.m. (n=25 injuries (WT);n=11 injuries (PAR4−/−);n=8 injuries (PAR4−/−with CRP+ADP)), wherens(nonsignificant)P>0.05,**P<0.005,***P<0.001.Pvalue was calculated by one-way ANOVA with Dunnett's post testing. Scale bar, 50 μm. Figure 2: Thrombin activation of platelets promotes leukocyte recruitment in vivo . C57BL/6J (WT) or PAR4 −/− mice were systemically administered DyLight 649 anti-GPIbβ Ab and PE-Gr-1 Ab before needle injury of mesenteric veins. ( a ) Thrombus surface area was quantified in the absence (no agonist) or presence of locally microinjected CRP and ADP (CRP/ADP), 20 min post injury as described in ‘Methods’. ( b ) Representative DIC images demonstrating thrombus instability in PAR4/mice as compared with C57BL/6J mice (WT) at the indicated times post injury (thrombus shaded in pink). ( c ) Leukocyte migration was quantified in the absence (no agonist) or presence of locally microinjected CRP and ADP (CRP/ADP), 20 min post injury as described in ‘Methods’. Results represent the mean±s.e.m. ( n =25 injuries ( WT ); n =11 injuries ( PAR4 −/− ); n =8 injuries ( PAR4 −/− with CRP+ADP)), where ns (nonsignificant) P >0.05, ** P <0.005, *** P <0.001. P value was calculated by one-way ANOVA with Dunnett's post testing. Scale bar, 50 μm. Full size image Provision of a P-selectin-positive surface is critical for leukocyte adhesion [34] , [35] . As thrombin can stimulate both endothelial cells and platelets to release P-selectin, the preceding results do not definitively distinguish between the activating effects of thrombin on platelets versus endothelial cells. To investigate this, we generated P-selectin BM chimeric mice with differential deletion of P-selectin from platelets ( Ly5.1 Recipient(R) /P-sel −/−BM ) or endothelial cells ( P-sel −/−R /Ly5.1 BM ; Fig. 3a–c ). Platelet thrombus formation was similar in all transplanted mouse cohorts following thrombin injection at the site of endothelial injury ( Fig. 3c ). However, leukocyte recruitment responses revealed a major role for platelet P-selectin in this process ( Fig. 3 ). While endothelial P-selectin alone ( Ly5.1 R /P-sel −/−BM ) was able to support a minor degree of leukocyte adhesion and migration on thrombi, platelet P-selectin ( Ly5.1 BM /P-sel −/−R ) played a more important role in enabling leukocyte–thrombus interactions ( Fig. 3a,b ). To confirm that platelets were playing the dominant role in promoting leukocyte recruitment and migration, we depleted platelets from mice and examined leukocyte recruitment and migration following thrombin microinjections at sites of endothelial needle injury. These findings confirmed that in the absence of platelets, injured endothelial cells were inefficient at promoting leukocyte recruitment ( Supplementary Fig. 2 ) and intravascular migration ( Fig. 3a–c ). Overall, these results demonstrate that thrombin induces rapid and efficient recruitment of leukocytes to sites of endothelial injury primarily through the activation of platelets. 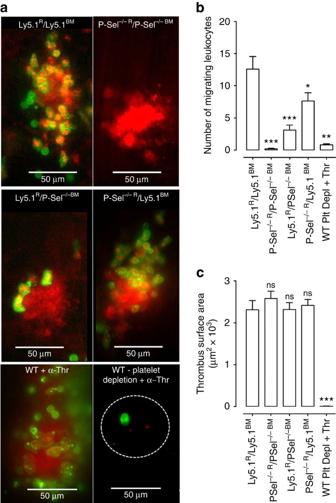Figure 3: Platelet P-selectin supports leukocyte recruitment to sites of vascular injury. Chimeric mice deficient in either endothelial or platelet P-selectin (P-sel) were generated by reconstitution of lethally irradiated wild-type (Ly5.1) orP-sel−/−recipient (R) mice with Ly5.1 orP-sel−/−BM. Four independent cohorts of chimeric mice were generated for these studies, including wild type (Ly5.1R/Ly5.1BM), platelet/endothelialP-sel−/−(P-sel−/−R/P-sel−/−BM), platelet-onlyP-sel−/−(Ly5.1R/P-sel−/−BM) and endothelial-onlyP-sel−/−(P-sel−/−R/Ly5.1BM). Mice from each cohort, C57BL/6J (WT) and mice with platelet depletion were injected with PE-anti-Gr-1 Ab (green) and DiOC6 (red) to visualize leukocyte and platelets, respectively, before needle injury of mesenteric veins and local microinjection of α-thrombin. (a) Representative epifluorescence images of leukocyte–thrombus interactions. Note—the area in platelet-depleted mice (right image) is demarcated by a dotted line. In the presence of platelets (left image), the platelet thrombus (red) extends well beyond the site of initial injury (IX81 Olympus, × 40 lens). (b,c) Quantification of the number of leukocytes undergoing directed migration towards the site of injury and (c) thrombus surface area (DIC microscopy). Results represent mean±s.e.m. (n=24 (Ly5.1R/Ly5.1BM), 23 (P-sel−/− R/P-sel−/− BM), 12 (Ly5.1R/P-sel−/− BM), 16 (P-sel−/− R/Ly5.1BM), 6 (WT+platelet depletion+α-thrombin microinjection)), wherensP>0.05, *P<0.05,**P<0.005,***P<0.001.Pvalue was calculated by one-way ANOVA with Dunnett's post testing. Scale bar, 50 μm. Figure 3: Platelet P-selectin supports leukocyte recruitment to sites of vascular injury. Chimeric mice deficient in either endothelial or platelet P-selectin (P-sel) were generated by reconstitution of lethally irradiated wild-type (Ly5.1) or P-sel −/− recipient (R) mice with Ly5.1 or P-sel −/− BM. Four independent cohorts of chimeric mice were generated for these studies, including wild type ( Ly5.1 R /Ly5.1 BM ), platelet/endothelial P-sel −/− ( P-sel −/−R /P-sel −/−BM ), platelet-only P-sel −/− ( Ly5.1 R /P-sel −/−BM ) and endothelial-only P-sel −/− ( P-sel −/−R /Ly5.1 BM ). Mice from each cohort, C57BL/6J ( WT ) and mice with platelet depletion were injected with PE-anti-Gr-1 Ab (green) and DiOC6 (red) to visualize leukocyte and platelets, respectively, before needle injury of mesenteric veins and local microinjection of α-thrombin. ( a ) Representative epifluorescence images of leukocyte–thrombus interactions. Note—the area in platelet-depleted mice (right image) is demarcated by a dotted line. In the presence of platelets (left image), the platelet thrombus (red) extends well beyond the site of initial injury (IX81 Olympus, × 40 lens). ( b , c ) Quantification of the number of leukocytes undergoing directed migration towards the site of injury and ( c ) thrombus surface area (DIC microscopy). Results represent mean±s.e.m. ( n =24 ( Ly5.1 R /Ly5.1 BM ), 23 ( P-sel −/− R /P-sel −/− BM ), 12 ( Ly5.1 R /P-sel −/− BM ), 16 ( P-sel −/− R /Ly5.1 BM ), 6 (WT+platelet depletion+α-thrombin microinjection)), where ns P >0.05, * P <0.05, ** P <0.005, *** P <0.001. P value was calculated by one-way ANOVA with Dunnett's post testing. Scale bar, 50 μm. Full size image Thrombin-binding interactions regulate leukocyte trafficking In addition to cleaving PARs, thrombin is rapidly incorporated into the body of thrombi through specific binding interactions with platelet GPIbα and fibrin. The impact of these binding interactions on leukocyte–thrombus interactions is unknown. α-thrombin blocked in the active site by PPACK (Phe-Pro-Arg-chloromethylketone; PPACK-α-thrombin) can completely displace catalytically active α-thrombin bound to the surface of platelets [36] , and in control experiments we confirmed competition between α-thrombin and PPACK-α-thrombin binding to platelets ( Supplementary Fig. 3 ). Notably, localized PPACK-α-thrombin injections at sites of needle injury in mesenteric veins resulted in the formation of large platelet thrombi ( Fig. 4a,b ), similar in magnitude to those observed with locally injected catalytically active α-thrombin. Additionally, thrombi formed after PPACK-α-thrombin injection were more efficient at recruiting leukocytes and directing their migration through the thrombus towards the site of endothelial injury ( Fig. 4a,c ). 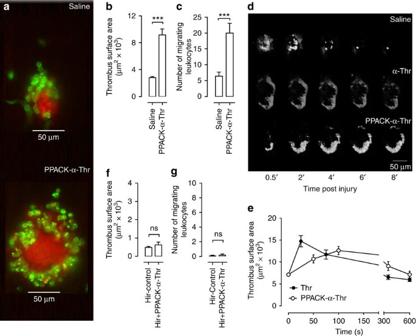Figure 4: Displacing bound thrombin enhances platelet and leukocyte recruitment. C57BL/6J mice were systemically injected with DiOC6 and PE-anti-Gr-1 Ab to monitor thrombus formation and leukocyte migration, respectively. Where indicated, hirudin (Hir—50 mg kg−1, to eliminate thrombin) or Alexa 488-anti-fibrin Ab (to monitor fibrin formation) were also administered systemically. All systemic administration was performed before needle injury, and immediately followed by local microinjection of either saline, thrombin (Thr) or PPACK-α-thrombin (PPACK α-Thr). Platelet thrombus formation and leukocyte migration were monitored using epifluorescence and DIC microscopy, as described under ‘Methods’. (a–c) Injury with microinjection of saline, α-thrombin or PPACK-α-thrombin. (a) Representative images demonstrating thrombus formation (red) and leukocyte recruitment/migration (green). (b) Quantification of thrombus surface area and (c) number of migrating leukocytes. Results represent mean±s.e.m., wheren=28 injuries (saline) andn=20 injuries (PPACK-α-thrombin). Note: quantification reflects the number of migrating leukocytes, not the total number of leukocytes recruited by the thrombus. (d) Fibrin formation (white) was monitored at the indicated times post injury using confocal microscopy (Nikon A1R confocal microscope, × 40 lens). 3D confocal images are from one experiment, representative of three independent experiments. (e) Thrombus surface area was quantified over 10 min following microinjection of the indicated agonist. Note—the delay in thrombus growth in PPACK-α-thrombin-injected mice compared with thrombin-injected mice. (f,g) Injury with microinjection of vehicle or PPACK-α-thrombin, in the presence of hirudin. Quantification of thrombus surface area (f) and number of migrating leukocytes (g) in hirudin-treated mice, with results representing mean±s.e.m. (n=11 injuries (Hir-Control),n=6 injuries (Hir-PPACK-α-Thr), wherensP>0.05,***P<0.001).Pvalue was calculated by unpaired Student’st-test. Scale bar, 50 μm. Figure 4: Displacing bound thrombin enhances platelet and leukocyte recruitment. C57BL/6J mice were systemically injected with DiOC6 and PE-anti-Gr-1 Ab to monitor thrombus formation and leukocyte migration, respectively. Where indicated, hirudin (Hir—50 mg kg −1 , to eliminate thrombin) or Alexa 488-anti-fibrin Ab (to monitor fibrin formation) were also administered systemically. All systemic administration was performed before needle injury, and immediately followed by local microinjection of either saline, thrombin (Thr) or PPACK-α-thrombin (PPACK α-Thr). Platelet thrombus formation and leukocyte migration were monitored using epifluorescence and DIC microscopy, as described under ‘Methods’. ( a – c ) Injury with microinjection of saline, α-thrombin or PPACK-α-thrombin. ( a ) Representative images demonstrating thrombus formation (red) and leukocyte recruitment/migration (green). ( b ) Quantification of thrombus surface area and ( c ) number of migrating leukocytes. Results represent mean±s.e.m., where n =28 injuries (saline) and n =20 injuries (PPACK-α-thrombin). Note: quantification reflects the number of migrating leukocytes, not the total number of leukocytes recruited by the thrombus. ( d ) Fibrin formation (white) was monitored at the indicated times post injury using confocal microscopy (Nikon A1R confocal microscope, × 40 lens). 3D confocal images are from one experiment, representative of three independent experiments. ( e ) Thrombus surface area was quantified over 10 min following microinjection of the indicated agonist. Note—the delay in thrombus growth in PPACK-α-thrombin-injected mice compared with thrombin-injected mice. ( f , g ) Injury with microinjection of vehicle or PPACK-α-thrombin, in the presence of hirudin. Quantification of thrombus surface area ( f ) and number of migrating leukocytes ( g ) in hirudin-treated mice, with results representing mean±s.e.m. ( n =11 injuries (Hir-Control), n =6 injuries (Hir-PPACK-α-Thr), where ns P >0.05, *** P <0.001). P value was calculated by unpaired Student’s t -test. Scale bar, 50 μm. Full size image To provide additional evidence that PPACK-α-thrombin enhanced platelet and leukocyte accumulation by displacing endogenously generated α-thrombin from one or more binding sites, we examined fibrin generation following PPACK-α-thrombin injection at sites of endothelial needle injury. As demonstrated in Fig. 4d , localized PPACK-α-thrombin injection greatly enhanced the intensity of anti-fibrin antibody bound around the margins of thrombi, suggesting that more fibrin fibrils were formed. However, time course studies revealed that fibrin formation and platelet thrombus growth were significantly delayed following PPACK-α-thrombin as compared with α-thrombin injection alone ( Fig. 4d,e ). This finding is consistent with the notion that PPACK-α-thrombin acts indirectly causing the time-dependent displacement of α-thrombin from binding sites. Moreover, in mice pretreated with the direct thrombin inhibitor hirudin, at concentrations that effectively blocked thrombin activity in vivo (50 mg kg −1 ), PPACK-α-thrombin failed to influence platelet recruitment and leukocyte migration ( Fig. 4f,g ). Taken together, these findings are consistent with an indirect effect of PPACK-α-thrombin enhancing the functional availability of endogenously generated α-thrombin. Thrombin-binding to GPIbα modulates leukocyte trafficking To provide direct experimental evidence that the binding of thrombin to GPIbα regulates thrombin’s ability to modulate leukocyte trafficking, we developed a mouse model in which endogenous platelet GPIbα is replaced by the human counterpart with the wild-type (WT) sequence ( h-GPIbα WT ) or with the D277N mutation ( h-GPIbα D277N ). Aspartic acid residue 277 was chosen for mutation as crystallographic [23] , [24] and functional [24] studies have revealed that the carboxyl group of this residue in human GPIbα is essential for measurable α-thrombin interaction. In control studies, we confirmed that platelet surface expression of h-GPIbα, as well as circulating platelet count and size, were similar in h-GPIbα WT and h-GPIbα D277N mice. Furthermore, the binding of human von Willebrand Factor (VWF) to h-GPIbα WT and h-GPIbα D277N platelets was indistinguishable (a detailed characterization of these mice will be reported elsewhere). In contrast, while α-thrombin binding to h-GPIbα WT platelets was preserved, there was no detectable α-thrombin binding to h-GPIbα D277N platelets ( Fig. 5a ). Analysis of platelet thrombus formation and leukocyte responses at sites of endothelial injury in the h-GPIbα D277N mouse revealed that both were enhanced relative to the h-GPIbα WT control ( Fig. 5b ). Notably, differences in platelet recruitment and leukocyte migration between h-GPIbα D277N and h-GPIbα WT mice could be overcome by the localized microinjection of exogenous α-thrombin ( Fig. 5c ), suggesting that the effect of eliminating thrombin binding to GPIbα in the mouse was to enhance the platelet-activating properties of the endogenously generated protease. 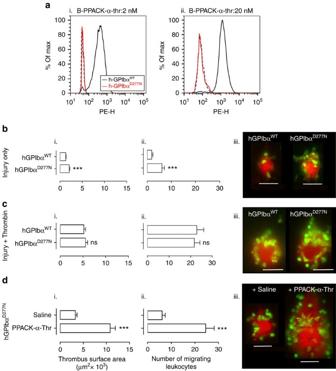Figure 5: Thrombin–GPIb interaction modulates platelet and leukocyte recruitment. (a) Quantification of biotin-labelled PPACK-α-thrombin (B-PPACK-α-thr) binding to platelets isolated fromh-GPIbαWT(black lines) orh-GPIbαD277N(red lines) mice, performed using flow cytometry as described under ‘Methods’. B-PPACK-α-thrombin was added at the indicated concentrations, followed by S-PE, with non-biotinylated PPACK-α-thrombin binding toh-GPIbαWTplatelets used as a negative control (black dotted lines). Histograms are taken from one experiment representative of three independent experiments (geometric mean fluorescence intensity measurements of PPACK-α-thrombin binding toh-GPIbαWTandh-GPIbαD277N: 2 nM PPACK-α-thrombin=602±124 and 24±2; 20 nM PPACK-α-thrombin=1,150±78 and 40±4 (mean±s.d.,n=3)). (b–d)hGPIbαWT(b,c) orhGPIbαD277N(d) mice were injected with a fluorescently labelled anti-Gr-1 Ab and DiOC6, before needle puncture of mesenteric veins. Thrombus surface area (i) and number of leukocytes migrating to sites of injury (ii) during a 20-min period immediately post injury/microinjection were monitored using epifluorescence or DIC microscopy. Representative images of thrombi (red) and associated leukocyte recruitment and migration (green) are depicted in iii. Platelet/leukocyte responses were monitored following injury alone (b), or injury plus local microinjection of α-thrombin (c) or PPACK-α-thrombin (d). Results represent the mean±s.e.m. ((b) injury only—n=24 injuries (hGPIbαWT),n=25 injuries (hGPIbαD277N); (c)injury+α-thrombin—n=17–18 injuries (hGPIbαWT),n=18–23 injuries (hGPIbαD277N); (d)injury+PPACK-α-thrombin—n=21–24 injuries (saline),n=17–30 injuries (PPACK-α-thrombin)), where ns, not significant;***P<0.001.Pvalue was calculated by unpaired Student’st-test. Note: the scale of theyaxis is kept consistent for all mouse genotypes to allow direct comparison. Scale bar, 50 μm. Figure 5: Thrombin–GPIb interaction modulates platelet and leukocyte recruitment. ( a ) Quantification of biotin-labelled PPACK-α-thrombin (B-PPACK-α-thr) binding to platelets isolated from h-GPIbα WT (black lines) or h-GPIbα D277N (red lines) mice, performed using flow cytometry as described under ‘Methods’. B-PPACK-α-thrombin was added at the indicated concentrations, followed by S-PE, with non-biotinylated PPACK-α-thrombin binding to h-GPIbα WT platelets used as a negative control (black dotted lines). Histograms are taken from one experiment representative of three independent experiments (geometric mean fluorescence intensity measurements of PPACK-α-thrombin binding to h-GPIbα WT and h-GPIbα D277N : 2 nM PPACK-α-thrombin=602±124 and 24±2; 20 nM PPACK-α-thrombin=1,150±78 and 40±4 (mean±s.d., n =3)). ( b – d ) hGPIb α WT ( b , c ) or hGPIb α D277N ( d ) mice were injected with a fluorescently labelled anti-Gr-1 Ab and DiOC6, before needle puncture of mesenteric veins. Thrombus surface area (i) and number of leukocytes migrating to sites of injury (ii) during a 20-min period immediately post injury/microinjection were monitored using epifluorescence or DIC microscopy. Representative images of thrombi (red) and associated leukocyte recruitment and migration (green) are depicted in iii. Platelet/leukocyte responses were monitored following injury alone ( b ), or injury plus local microinjection of α-thrombin ( c ) or PPACK-α-thrombin ( d ). Results represent the mean±s.e.m. (( b ) injury only— n =24 injuries ( hGPIb α WT ), n =25 injuries ( hGPIb α D277N ); ( c ) injury+ α- thrombin — n =17–18 injuries ( hGPIb α WT ), n =18–23 injuries ( hGPIb α D277N ); ( d ) injury+PPACK -α- thrombin — n =21–24 injuries (saline), n =17–30 injuries (PPACK-α-thrombin)), where ns, not significant; *** P <0.001. P value was calculated by unpaired Student’s t -test. Note: the scale of the y axis is kept consistent for all mouse genotypes to allow direct comparison. Scale bar, 50 μm. Full size image On the basis of the results presented above, we used the h-GPIbα D277N mouse model to investigate whether the effects of PPACK-α-thrombin on platelet recruitment and leukocyte migration towards sites of endothelial injury were solely dependent on the displacement of endogenous α-thrombin bound to GPIbα. If this were the case, PPACK-α-thrombin, which cannot bind to h-GPIbα D277N platelets, would have no effect on the responses to endothelial injury in h-GPIbα D277N mice. To the contrary, microinjected PPACK-α-thrombin markedly enhanced platelet thrombus size and leukocyte migratory responses in h-GPIbα D277N mouse veins following needle injury ( Fig. 5d ). This enhanced thrombotic response induced by PPACK-α-thrombin indicates that other thrombin-binding partners, such as fibrin, may play an important role in regulating α-thrombin’s thromboinflammatory effects. Fibrinolysis abolishes prothrombotic effects of PPACK-thrombin Fibrin binds α-thrombin in a low affinity, high-capacity manner and the binding of α-thrombin to fibrin and fibrinogen is important for reducing the prothrombotic effects of the protease [37] , [38] . To investigate whether the enhancing effects of PPACK-α-thrombin on the recruitment of platelets and leukocytes to sites of endothelial injury were fibrin-dependent, we lysed fibrin polymers by infusing recombinant t-PA (rt-PA) systemically into mice up to 3 h after the formation of platelet- and fibrin-rich thrombi in mesenteric veins. Fibrinolysis induced by rt-PA markedly reduced thrombus size ( Fig. 6a ) even after fibrin generation and platelet stimulation was enhanced by local α-thrombin injection ( Fig. 6a ). After fibrin lysis, platelets were no longer responsive to localized PPACK-α-thrombin microinjection, whereas responsiveness to α-thrombin remained intact ( Fig. 6b ). These results support the concept that the effect of PPACK-α-thrombin on the platelet response to vascular injury is critically dependent on fibrin. 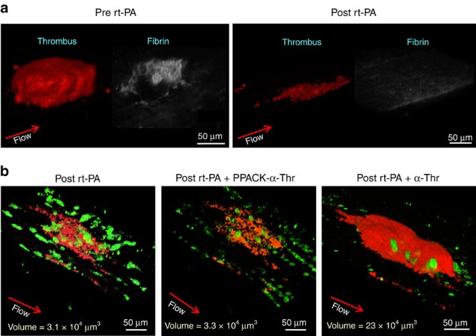Figure 6: Effect of PPACK-thrombin on platelets and leukocytes is fibrin-dependent. C57BL/6J mice were injected with Alexa 488-anti-fibrin Ab, PE-conjugated anti-Gr-1 Ab and DyLight 649 anti-GPIbβ Ab before needle injury of mesenteric veins followed by local microinjection of α-thrombin (1.4 nl boluses of 100 U ml−1, about five cycles), to allow the development of a platelet thrombus. After 1.5–3 h injury/thrombin administration, mice were systemically administered recombinant t-PA (2 mg kg−1bolus and 36 mg kg−1per hour infusion for 30 min). Platelet thrombus formation, fibrin formation and leukocyte migration were monitored using confocal microscopy. (a) Representative 3D images demonstrating platelets (thrombi) alone (red), fibrin alone (white) 1.5–3 h post-needle injury, pre- and post-rt-PA infusion. (b) Representative 3D images of thrombi and leukocyte recruitment post rt-PA infusion alone (post-rt-PA) or post-rt-PA followed by a second local microinjection of either α-thrombin (α-Thr) or PPACK-α-thrombin (PPACK-α-Thr; platelets: red; leukocytes: green). The resultant thrombus volume post rt-PA alone or post-second microinjection of α-thrombin/PPACK-α-thrombin was quantitated as detailed under Methods. Note—thrombus growth following the injection of α-thrombin but not PPACK-α-thrombin. Scale bar, 50 μm. Figure 6: Effect of PPACK-thrombin on platelets and leukocytes is fibrin-dependent. C57BL/6J mice were injected with Alexa 488-anti-fibrin Ab, PE-conjugated anti-Gr-1 Ab and DyLight 649 anti-GPIbβ Ab before needle injury of mesenteric veins followed by local microinjection of α-thrombin (1.4 nl boluses of 100 U ml −1 , about five cycles), to allow the development of a platelet thrombus. After 1.5–3 h injury/thrombin administration, mice were systemically administered recombinant t-PA (2 mg kg −1 bolus and 36 mg kg −1 per hour infusion for 30 min). Platelet thrombus formation, fibrin formation and leukocyte migration were monitored using confocal microscopy. ( a ) Representative 3D images demonstrating platelets (thrombi) alone (red), fibrin alone (white) 1.5–3 h post-needle injury, pre- and post-rt-PA infusion. ( b ) Representative 3D images of thrombi and leukocyte recruitment post rt-PA infusion alone (post-rt-PA) or post-rt-PA followed by a second local microinjection of either α-thrombin (α-Thr) or PPACK-α-thrombin (PPACK-α-Thr; platelets: red; leukocytes: green). The resultant thrombus volume post rt-PA alone or post-second microinjection of α-thrombin/PPACK-α-thrombin was quantitated as detailed under Methods. Note—thrombus growth following the injection of α-thrombin but not PPACK-α-thrombin. Scale bar, 50 μm. Full size image Fibrin acts as a physical barrier to leukocyte migration A notable consequence of rt-PA-induced fibrinolysis was the marked increase in number of leukocytes that were able to migrate to the initial site of injury in the centre of the thrombus ( Fig. 7a ). Quantitative analysis revealed that following fibrinolysis there was an approximately fourfold increase in the number of leukocytes migrating to the site of endothelial injury ( Fig. 7b ). Moreover, there was more extensive migration of leukocytes into the extravascular space following fibrinolysis ( Fig. 7c ), suggesting a potentially important role for fibrin in retarding the migration of leukocytes to sites of vessel wall injury. 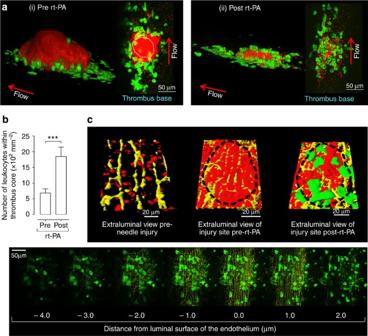Figure 7: Fibrinolysis promotes leukocyte migration to sites of vascular injury. C57BL/6J mice were injected with antibodies, vessel injury initiated and rt-PA infused, as described forFig. 6. (a) Representative 3D (left, i,ii) and 2D (right, i,ii) images illustrating different leukocyte (green)-migratory behaviour pre- and 30 min post-rt-PA infusion at the thrombus base (red). Note—leukocyte migration was limited to the periphery of the thrombus pre-rt-PA infusion, but continued throughout the body of the thrombus post-rt-PA infusion. These images are representative of four independent experiments (38 thrombi). (b) Quantification of the number of leukocytes migrating into the thrombus core, pre- and post-rt-PA infusion. Results represent the mean±s.e.m. (n=10 mice, 57 thrombi (pre-rt-PA);n=4 mice, 38 thrombi (post-rt-PA)), where***P<0.001. Pvalue was calculated by unpaired Student’st-test. (c) Lower panel—representative confocal sections demonstrating leukocytes from 4 μm below the endothelial surface (−4.0) to 2 μm above (2.0) the endothelial surface, and leukocyte (green) migration from intra- to extraluminal surface at the site of vessel injury post-rt-PA infusion. Upper panel—representative images of extraluminal view of mesenteric veins pre- and post-needle injury (black broken line) and following rt-PA infusion to illustrate leukocyte (green) migration to the extraluminal side of the vessel post-rt-PA infusion. Note—collagen fibres, yellow; platelets, red; area of vessel injury, broken line. Scale bar, 50 or 20 μm as indicated in figure. Figure 7: Fibrinolysis promotes leukocyte migration to sites of vascular injury. C57BL/6J mice were injected with antibodies, vessel injury initiated and rt-PA infused, as described for Fig. 6 . ( a ) Representative 3D (left, i,ii) and 2D (right, i,ii) images illustrating different leukocyte (green)-migratory behaviour pre- and 30 min post-rt-PA infusion at the thrombus base (red). Note—leukocyte migration was limited to the periphery of the thrombus pre-rt-PA infusion, but continued throughout the body of the thrombus post-rt-PA infusion. These images are representative of four independent experiments (38 thrombi). ( b ) Quantification of the number of leukocytes migrating into the thrombus core, pre- and post-rt-PA infusion. Results represent the mean±s.e.m. ( n =10 mice, 57 thrombi (pre-rt-PA); n =4 mice, 38 thrombi (post-rt-PA)), where *** P <0.001 . P value was calculated by unpaired Student’s t -test. ( c ) Lower panel—representative confocal sections demonstrating leukocytes from 4 μm below the endothelial surface (−4.0) to 2 μm above (2.0) the endothelial surface, and leukocyte (green) migration from intra- to extraluminal surface at the site of vessel injury post-rt-PA infusion. Upper panel—representative images of extraluminal view of mesenteric veins pre- and post-needle injury (black broken line) and following rt-PA infusion to illustrate leukocyte (green) migration to the extraluminal side of the vessel post-rt-PA infusion. Note—collagen fibres, yellow; platelets, red; area of vessel injury, broken line. Scale bar, 50 or 20 μm as indicated in figure. Full size image To investigate the impact of fibrin on leukocyte migration, we compared the velocity of migrating leukocytes under experimental conditions promoting platelet thrombus formation with high levels of fibrin—that is, localized α-thrombin injection at sites of needle injury—with platelet thrombi generated in the absence of fibrin. These latter conditions involved pretreating mice with high-dose hirudin (50 mg kg −1 ; to eliminate α-thrombin catalytic function) while activating platelets at sites of needle injury with microinjected CRP and PAR4 agonist peptide. This resulted in the formation of stable platelet aggregates that efficiently recruited leukocytes ( Supplementary Fig. 3 ). Measurement of individual neutrophil migration velocities revealed no difference in velocity at the initiation of migration in thrombin-stimulated versus fibrin-free thrombi ( Fig. 8a ). In contrast, after 10 min of migration, neutrophils were almost stationary in thrombin-stimulated thrombi, whereas in fibrin-free thrombi the velocity of individual migrating leukocytes was ∼ 4.2 μm min −1 ( Fig. 8a ), providing further support for the concept that fibrin plays an important role in the regulation of leukocyte migration. 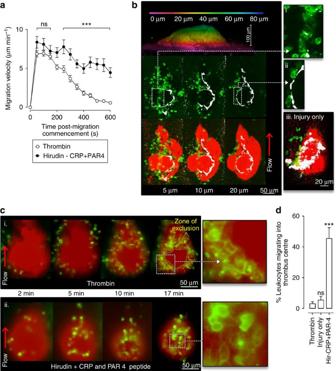Figure 8: Fibrin impedes leukocyte migration. C57BL/6J mice were administered Alexa 488-anti-fibrin Ab, DyLight 649 anti-GPIbβ Ab (a,b), or PE-anti-Gr-1 Ab and DiOC6 (c,d) and hirudin (50 mg kg−1), where indicated, before needle injury of mesenteric veins. Resultant thrombi were enhanced through local microinjection of thrombin (a—open symbols;b—i,ii,c—i) or a combination of CRP- and PAR4-activating peptide (a—solid symbols;c—ii, in the case of hirudin-treated mice). Thrombus formation, leukocyte migration and fibrin accumulation were monitored/analysed using epifluorescence and confocal microscopy, as described under ‘Methods’. (a) Quantification of migration velocity of individual leukocytes traversing thrombi, 10 min after initiation of migration. Results represent mean±s.e.m. (n=27 (thrombin);n=50 (hirudin, CRP/PAR4)). (b) Top panel—representative 3D image of a thrombus withz-depth (height) colour coding. Middle/lower panels—representative two-dimensional (2D) images depicting leukocyte migratory behaviour (green), fibrin deposition (white) and platelet adhesion (red; lower panel only) on a representative thrombus, acquired at the indicated distances from the thrombus base. Note insets (i–iii)—migrating leukocytes breach the thrombus core in areas devoid of fibrin (i), while migration into the core is restricted by an intact fibrin ring (ii). Fibrin formation and fibrin restriction of leukocyte migration are not limited to thrombin-treated thrombi and also occur following needle injury alone (iii). (c) Representative images demonstrating leukocyte migration (green) through control thrombi (red) microinjected with thrombin (i) or thrombi formed in the presence of hirudin and microinjected with CRP/PAR4 (ii). Note—a zone of exclusion (yellow broken line) preventing leukocyte migration into the core is present only in thrombin, (i) but not in hirudin+CRP/PAR4 agonist peptide (ii)-injected thrombi. (d) Quantification of the number of leukocytes migrating into the thrombus core in the presence or absence (Hirudin+CRP/PAR4 peptide) of thrombin. Results represent mean±s.e.m. (n=9 injuries) wherensP>0.05;***P<0.001. Pvalue calculated using unpaired Student’st-test inaand one-way ANOVA with Dunnett’s post-testing ind. Scale bar, 50 or 20 μm as indicated in figure. Figure 8: Fibrin impedes leukocyte migration. C57BL/6J mice were administered Alexa 488-anti-fibrin Ab, DyLight 649 anti-GPIbβ Ab ( a , b ), or PE-anti-Gr-1 Ab and DiOC6 ( c , d ) and hirudin (50 mg kg −1 ), where indicated, before needle injury of mesenteric veins. Resultant thrombi were enhanced through local microinjection of thrombin ( a —open symbols; b —i,ii, c —i) or a combination of CRP- and PAR4-activating peptide ( a —solid symbols; c —ii, in the case of hirudin-treated mice). Thrombus formation, leukocyte migration and fibrin accumulation were monitored/analysed using epifluorescence and confocal microscopy, as described under ‘Methods’. ( a ) Quantification of migration velocity of individual leukocytes traversing thrombi, 10 min after initiation of migration. Results represent mean±s.e.m. ( n =27 (thrombin); n =50 (hirudin, CRP/PAR4)). ( b ) Top panel—representative 3D image of a thrombus with z -depth (height) colour coding. Middle/lower panels—representative two-dimensional (2D) images depicting leukocyte migratory behaviour (green), fibrin deposition (white) and platelet adhesion (red; lower panel only) on a representative thrombus, acquired at the indicated distances from the thrombus base. Note insets (i–iii)—migrating leukocytes breach the thrombus core in areas devoid of fibrin ( i ), while migration into the core is restricted by an intact fibrin ring (ii). Fibrin formation and fibrin restriction of leukocyte migration are not limited to thrombin-treated thrombi and also occur following needle injury alone (iii). ( c ) Representative images demonstrating leukocyte migration (green) through control thrombi (red) microinjected with thrombin ( i ) or thrombi formed in the presence of hirudin and microinjected with CRP/PAR4 (ii). Note—a zone of exclusion (yellow broken line) preventing leukocyte migration into the core is present only in thrombin, ( i ) but not in hirudin+CRP/PAR4 agonist peptide (ii)-injected thrombi. ( d ) Quantification of the number of leukocytes migrating into the thrombus core in the presence or absence (Hirudin+CRP/PAR4 peptide) of thrombin. Results represent mean±s.e.m. ( n =9 injuries) where ns P >0.05; *** P <0.001 . P value calculated using unpaired Student’s t -test in a and one-way ANOVA with Dunnett’s post-testing in d . Scale bar, 50 or 20 μm as indicated in figure. Full size image To investigate the possibility that fibrin was forming a physical barrier to leukocyte migration, confocal microscopy was performed to examine the impact of fibrin distribution on the kinetics of leukocyte migration. Microinjection of α-thrombin resulted in the formation of a fibrin ring around the outer margins of platelet thrombi ( Fig. 8b ). Real-time imaging of leukocytes revealed that migration was completely halted at the fibrin ring, with substantial intrathrombus migration only observed in regions of the thrombus devoid of detectable fibrin ( Fig. 8bi , Supplementary Movie 1 ), which provides a likely explanation for marked reduction, but not complete absence of leukocytes seen in the centre of the thrombus core preceding fibrinolysis. Leukocyte migration was similarly restrained by the presence of fibrin in a model of repetitive needle injury alone, independent of thrombin injection ( Fig. 8biii and Supplementary Movie 2 ), indicating that the barrier function of fibrin occurs as a general feature of vascular injury. In contrast to the restricted leukocyte migratory response imposed by fibrin ( Fig. 8ci and Supplementary Movie 1 ), leukocytes migrated through the entire body of fibrin-free thrombi formed by platelets activated by CRP and PAR4 agonist peptide in hirudin-treated mice ( Fig. 8cii , Supplementary Fig. 4 and Supplementary Movie 1 ). Relative to thrombin-treated thrombi, there was a greater than 15-fold increase in the number of leukocytes migrating into the central region of the thrombus at the initial site of injury in fibrin-free thrombi ( Fig. 8d ). Analysis of individual migrating leukocytes revealed that all cells freely crawled around the periphery of the fibrin barrier, engaging fibrin in a dynamic and highly motile manner. None of the leukocytes formed stable adhesive contacts with fibrin polymers, suggesting that fibrin was primarily forming a ‘barrier’ function rather than restraining migration by acting as an adhesive substrate. The studies presented here define a series of molecular events, initiated by coagulation activation with α-thrombin generation, regulating leukocyte trafficking at sites of endothelial injury ( Fig. 9 ). Among these, thrombin-dependent cleavage of platelet PAR4 is crucial for leukocyte recruitment and migration to sites of endothelial perturbation. This process appears to be subjected to spatial and temporal regulation by the two major thrombin-binding partners present in thrombi, GPIbα and fibrin. GPIbα, by binding α-thrombin with high affinity, can reduce platelet activation and early leukocyte recruitment. Progressive fibrin deposition then controls further accumulation and migration of recruited leukocytes, with a mechanism balanced by activation of fibrinolysis. Thus, through distinct molecular interactions, thrombin both promotes and retards leukocyte trafficking, suggesting that targeting thrombin’s specific molecular interactions, rather than global anticoagulant treatment, could modulate thromboinflammation with reduced impact on haemostasis. 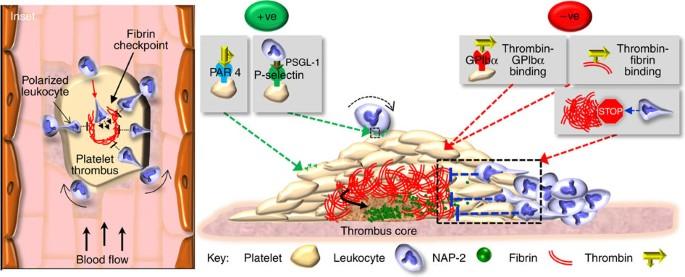Figure 9: Balanced thrombin interactions regulate leukocyte trafficking. Leukocyte migration during thromboinflammation is initiated and positively regulated (+ve) by thrombin-dependent recruitment of leukocytes to the surface of platelet thrombi via PAR4-dependent expression of platelet P-selectin. Leukocyte polarization and intravascular migration through the body of platelet thrombi is contingent on the development of a NAP-2 chemokine gradient32leading to circumferential migration through the body of the thrombus (inset—indicated by red arrow) rather than perpendicular crawling in the classical intravascular leukocyte-trafficking model. α-Thrombin binding to GPIbα and fibrin serves as a negative (−ve) regulators of leukocyte trafficking. The thrombin-binding function of both GPIbα and fibrin serves to limit the availability of catalytically active thrombin and prevent excessive thrombus formation and leukocyte recruitment. In addition, fibrin serves as a physical barrier to limit intravascular leukocyte migration to sites of endothelial injury (inset). Figure 9: Balanced thrombin interactions regulate leukocyte trafficking. Leukocyte migration during thromboinflammation is initiated and positively regulated (+ve) by thrombin-dependent recruitment of leukocytes to the surface of platelet thrombi via PAR4-dependent expression of platelet P-selectin. Leukocyte polarization and intravascular migration through the body of platelet thrombi is contingent on the development of a NAP-2 chemokine gradient [32] leading to circumferential migration through the body of the thrombus (inset—indicated by red arrow) rather than perpendicular crawling in the classical intravascular leukocyte-trafficking model. α-Thrombin binding to GPIbα and fibrin serves as a negative (−ve) regulators of leukocyte trafficking. The thrombin-binding function of both GPIbα and fibrin serves to limit the availability of catalytically active thrombin and prevent excessive thrombus formation and leukocyte recruitment. In addition, fibrin serves as a physical barrier to limit intravascular leukocyte migration to sites of endothelial injury (inset). Full size image Dysregulated blood coagulation, platelet activation and endothelial dysfunction are common features of a broad range of thromboinflammatory disorders, including ischaemia-reperfusion injury [39] , venous thromboembolism [40] , thrombotic microangiopathies [41] and transplant rejection [42] , [43] . The experimental needle injury method used in this study has enabled detailed insight into the mechanisms by which dysregulated thrombin generation on the surface of procoagulant endothelial cells may influence intravascular leukocyte trafficking in vivo . While this model is not designed to mimic the precise sequence of pathogenetic events linked to specific thromboinflammatory diseases, it nonetheless provides important insights into the molecular processes by which dying endothelial cells promote leukocyte trafficking in vivo . The disruption of membrane phospholipid asymmetry in endothelial cells leading to PS exposure is a characteristic feature of dying cells regardless of the cause [44] , [45] , as in the antiphospholipid syndrome [46] , in response to immunomodulatory and chemotherapeutic regimens containing agents such as thalidomide [47] and arsenic [48] , and after ischaemia reperfusion [49] , [50] , [51] . Therefore, our observations related to PS-positive endothelial cells after needle injury may have relevance to disease processes. Our studies, including PAR4 knockout, platelet-depleted and selective platelet or endothelial P-selectin-deficient mice, highlight the importance of thrombin-dependent platelet activation in promoting leukocyte recruitment to sites of endothelial injury. Indeed, even localized thrombin injection with direct stimulation of endothelial cells is inefficient at promoting rapid and sustained leukocyte adhesion in the absence of platelets. While these findings demonstrate a major role for platelet PAR4 in promoting leukocyte recruitment in our endothelial injury model, PARs’ contributions to thromboinflammatory responses such as ischaemia-reperfusion injury remain controversial. Some studies have suggested that PAR activation is critical for ischaemia-reperfusion-induced organ injury [52] ; however, others failed to identify a role of PARs in linking coagulation with inflammation [53] . Such discordant conclusions may reflect the variable influence of platelet activation on thromboinflammatory reactions in different experimental models. Of all the conditions we tested, microinjected thrombin was the most potent inducer of leukocyte recruitment [20] . While microinjection of specific agonists allows precise spatiotemporal control of platelet activation and fibrin formation, the possibility of overwhelming physiologic mechanisms is a potential limitation. Thus, we have titrated microinjected α-thrombin to obtain thrombus size and fibrin generation similar to those induced by PPACK-thrombin on the basis of the assumption that the effects of the latter reflect the activity of displaced endogenously generated thrombin following needle injury alone. Furthermore, all the conclusions involving PAR4, GPIb and fibrin have been confirmed in response to repetitive needle injury alone, reducing the likelihood that the processes analysed are primarily a feature of supraphysiological thrombin concentrations. The importance of low levels of thrombin in regulating leukocyte recruitment is supported by the studies in hGPIbα D277N mice, in which even a relatively mild vascular injury with low fibrin generation caused enhanced platelet and leukocyte responses. Abrogating the binding of α-thrombin to GPIbα, therefore, appears to increase the bioavailability of catalytically active thrombin, and is capable of enhancing platelet activation and leukocyte recruitment. It is noteworthy that with higher thrombin levels, either after severe endothelial needle injury or microinjection of thrombin or PPACK-thrombin, the relative contribution of GPIb-thrombin binding to the regulation of leukocyte migration was less obvious, with fibrin appearing to play a major role in regulating intravascular leukocyte trafficking. Thus, through thrombin’s distinct molecular interactions, principally involving GPIb and fibrin, the haemostatic system appears to have evolved mechanisms of limiting thrombin’s proinflammatory effects over a broad range of protease concentrations. The enhanced platelet response in hGPIb D277N mice contrasts with the impaired thrombus development reported in mice harbouring a different GPIb mutation ( hGPIb Y276F ) [54] but with similar effects on thrombin binding. While the reasons for the observed discrepancy are not immediately apparent, an explanation may be the use of an arterial thrombosis model with hGPIb Y276F mice as opposed to studies in the venous circulation in our case, with the possible contribution of different effects of the mutations on VWF binding and background strain differences. An unexpected finding in our study was the potency by which catalytically inactive PPACK-α-thrombin enhanced leukocyte recruitment to sites of endothelial injury likely by displacing endogenously generated thrombin from one or more thrombin-binding sites. The two major thrombin-binding sites within a developing thrombus are GPIbα and fibrin. The demonstration that locally injected PPACK-α-thrombin was able to augment platelet and leukocyte recruitment in hGPIb D277N mice indicated that thrombin-binding sites additional to GPIbα were likely to be important in limiting the recruitment of leukocytes to sites of endothelial injury. The demonstration that the effects of PPACK-α-thrombin were abrogated by pretreating mice with hirudin or through lysis of fibrin with rt-PA, suggests a potentially important role for fibrin in modulating the effects of thrombin on leukocyte recruitment. This ‘thrombin regulatory’ function of fibrin(ogen) is likely to be of pathophysiological relevance to humans as demonstrated by the predisposition to both venous and arterial thrombotic events in individuals with mutant fibrin(ogen)s that have reduced thrombin-binding capacity, including fibrinogen New York [38] and fibrinogen Naples I (ref. 55 ). Whether other thrombin-binding partners including antithrombin [56] , thrombomodulin, heparin cofactor II and glycosaminoglycans contribute to the modulation of thrombin’s proinflammatory functions remains to be explored. A limitation of our studies in mice is that they may not faithfully recapitulate the molecular interactions that are relevant to humans, as mice have a different complement of platelet PAR receptors [5] . Mouse platelets express PAR3 and PAR4 with the former serving as a cofactor for the latter. Human platelets, however, express PAR1 and PAR4, which signal independently but with different thresholds (higher in PAR4) for thrombin activation. In addition, GPIbα acts as a cofactor to enhance thrombin cleavage of PAR1 on intact platelets [57] . Therefore, predicting what the net effects of disrupting thrombin binding to GPIbα might be on leukocyte responses in humans is not straightforward. The reduced PAR1-mediated platelet activation at low thrombin concentrations could blunt the early response; however, this could be quickly compensated by increased PAR4-mediated leukocyte recruitment leading to an overall enhanced thromboinflammatory response as seen in the hGPIbα D277N mouse. A striking finding from our experimental model was the effect of rt-PA on leukocyte migration at sites of endothelial injury. Both clinical [58] and experimental [59] studies have revealed that neutrophil accumulation is a hallmark of ischaemia-reperfusion injury that occurs within hours of initiation of reperfusion. In addition, rt-PA has been shown to increase tissue injury and enhance neutrophil tissue infiltration following ischaemia-reperfusion injury to the brain [60] , lung [61] and kidneys [62] . The known proinflammatory function of recombinant t-PA has been partly attributed to its direct activating effects on the endothelium and inflammatory cells, as well as through the generation of fibrin degradation products [63] and plasmin [64] . In addition to these well-known proinflammatory effects, the studies presented here define an additional mechanism by which rt-PA may enhance thromboinflammatory responses by undermining the physical barrier function of fibrin on leukocyte migration. Such a finding may also help explain the reduced infiltration of tissues by leukocytes in mice administered rFXIII (refs 65 , 66 ). Whether therapeutic targeting of specific platelet chemokines to reduce intravascular leukocyte migration will reduce t-PA-dependent leukocyte infiltration remains an interesting possibility for future investigation. Reagents Anti-Gr-1(RB6–8C5)-phycoerythrin (PE) monoclonal antibody (Ab) and PECAM/CD31-FITC (Clone:390) Ab were from eBiosciences Inc. (CA, USA). Anti-GPIbα (R300) and anti-mouse GPIbβ-DyLight 488/649 Abs were from Emfret Analytics (Wurzburg, Germany). DiOC6 was sourced from Molecular Probes (Eugene, OR, USA). Anti-fibrin Ab (IgG1) was purified from murine hybridoma HB-8545 (American Type Culture Collection) maintained at The Scripps Research Institute; the Ab was labelled with Alexa Fluor 488. Annexin V was purchased from Sigma (St Louis, MO, USA) and was labelled with Alexa Fluor 488 or 546. Alteplase (rt-PA) was from Boehringer Ingelheim (Ingelheim, Germany). CRP was from Professor Richard Farndale (Biochemistry Department, Cambridge University, UK). Thrombin was purchased from Siemens Healthcare (Melbourne, Australia). PAR4 peptide was from Auspep (Melbourne, Australia). PPACK was from Haematologic Technologies Inc. (Essex Junction, VT, USA). PPACK-α-thrombin was produced by treating human (h) α-thrombin (Haematologic Technologies Inc.) with a 25-fold molar excess of PPACK for 8 h at 22–25 °C and 3 days at 4 °C as previously described [22] . Residual thrombin proteolytic activity was assessed by measuring the clotting time of a 4-mg ml −1 fibrinogen solution and confirmed to be <1:1,000,000 of untreated α-thrombin [22] . Mouse strains All procedures involving mice were approved by the Alfred Medical Research and Education Precinct Animal Ethics Committee (Melbourne, Australia), project numbers E/1002/2010/M and E/0937/2010/M. All intravital microscopy studies were performed on 5–6-week-old male mice with a body weight of 16–20 g for optimal imaging purposes. PAR4 −/− mice were from Professor Shaun Coughlin (University of California, San Francisco, CA, USA). P-selectin −/− mice were obtained from the Jackson Laboratory (CA, USA), while the Ly5.1 mice were sourced from the Walter and Eliza Hall Institute (WEHI-BBS, Kew, Victoria, Australia). Power calculations were used to establish sample size for in vivo animal experiments (significance level=0.01; statistical power set at 80%). If statistical significance was reached with fewer animals, no additional animals were utilized. Mice expressing human GPIbα within the mouse platelet GPIb-IX-V complex were generated at The Scripps Research Institute (CA, USA). Transgenic expression of WT human GPIbα ( h-GPIbα WT ) was achieved [67] using a 6-kb EcoRI DNA fragment containing the entire human GPIbα gene, including ∼ 2.5 kb of promoter sequence to support platelet-specific expression; the only difference was that we used C57BL/6J mouse zygotes. The same approach was used to generate a strain of mice expressing mutated human GPIbα. For this, we replaced the Asp277 codon with Asn ( h-GPIbα D277N ) in the same EcoRI DNA fragment. Replacement of the endogenous homologue with huGPIbα in mouse platelets was achieved as previously described [68] by crossing C57BL/6J GPIbα −/− and h-GPIbα WT or h-GPIbα D277N transgene-expressing mice. Expression of the human transgene in the absence of murine GPIbα was determined using flow cytometry, and mice with the desired phenotype were bred to establish colonies for experimental use. P-selectin chimeric mice were generated using 6-week-old WT Ly5.1 and P-selectin −/− male mice, both as donors and recipients in BM transplantation experiments to generate mice expressing P-selectin exclusively on endothelial cells or platelets. WT Ly5.1 mice transplanted with WT Ly5.1BM and P-selectin −/− mice transplanted with P-selectin −/− BM served as positive and negative controls, respectively. BM was harvested from the tibiae and femora of donor mice and cell counts were adjusted to 1.0 × 10 7 ml −1 using PBS. Recipient mice received total body irradiation given as two fractions of 550 rad, 3 h apart as BM transplantation conditioning. Donor BM (1 × 10 6 cells) was introduced to recipients via tail vein injection. Haematopoietic reconstitution was determined 8 weeks post transplant and assessed with the quantification of peripheral blood counts, as well as degree of chimerism by differential CD45 expression on circulating leukocytes using flow cytometry (PE-conjugated anti-CD45.1 (clone A20) and fluorescein isothiocyanate (FITC)-conjugated anti-CD45.2 (clone 104) antibodies, BD Pharmingen). Generation of biotin–PPACK and thrombin-binding studies Biotin–PPACK (B-PPACK) and human α-thrombin (FIIa; Haematologic Technologies Inc.) were mixed to block the active site of the protease (B-PPACK-α-thrombin) and characterized [22] . B-PPACK-α-thrombin at 2 or 20 nM was added to 2 × 10 7 ml −1 PGE 1 -treated washed mouse platelets and incubated for 15 min at room temperature (22–25 °C) in the presence of 0.1% fatty-acid-free bovine serum albumin (BSA-FAF; Sigma Aldrich, St Louis, MO, USA). PE-conjugated streptavidin (S-PE; premium grade, Invitrogen, Carlsbad, CA, USA) was added (0.5:1 molar ratio with biotin) and incubated for an additional 25 min with no further dilutions. The binding of S-PE-B-PPACK-α-thrombin to platelets was then evaluated with a LSRII flow cytometer (BD Bioscience, San Jose, CA, USA). The fluorescence intensity of 10,000 events was acquired with the FACSDiva software and analysed with FlowJo. To define the PPACK-α-thrombin inhibition mode, mathematical analysis of data was performed as described in legend for Supplementary Fig. 3 . Clotting time was measured in the presence of α-Thrombin 0.1 nM with or without a 1,000-fold molar excess of PPACK-α-thrombin and defined as absence of movement of a metal ball in a plastic cuvette incubated at 37 °C. Residual thrombin activity in the presence of PPACK-α-thrombin was calculated from a standard curve of clotting time in the absence of the inhibitor and residual thrombin activity was expressed as percentage of the original α-Thrombin concentration. For aggregation studies, aliquots of 0.4 ml of 2 × 10 8 ml −1 washed mouse platelets were placed in glass cuvettes and stirred with a Teflon-coated magnetic bar at 1,200 r.p.m. 37 °C, in an aggregometer (Chrono-Log Corp, PA, USA) connected to a personal computer through an analogue/digital signal converter. Platelet aggregation was measured by recording for 4 min the increase in light transmittance through the suspension induced by the addition of 1 nM α-Thrombin, in the presence of CaCl 2 2 mM with or without a 1,000-fold molar excess of PPACK-α-thrombin. Inhibition of thrombin activity was expressed as percentage of the maximal extent of aggregation in the presence of PPACK-a-thrombin relative to the maximal extent obtained without the inhibitor. Displacement of GPIbα-bound α-thrombin by PPACK-α-thrombin B-PPACK-α-thrombin was added to 2 × 10 7 ml −1 PGE 1 -treated mouse-washed platelets at the concentration of 1.5 nM, with or without catalytically active α-thrombin at different concentrations between 0.07 and 150 nM. These mixtures were incubated for 15 min at room temperature (22–25 °C) in the presence of 0.1% BSA-FAF (Sigma Aldrich), after which S-PE (premium grade; Invitrogen) was added (0.5:1 molar ratio with biotin) and incubated for an additional 25 min with no further dilutions. The amount of S-PE-B-PPACK-α-thrombin bound to platelets was then measured with flow cytometry using a LSRII flow cytometer (BD Bioscience); data were acquired with the FACSDiva software and analysed with FlowJo. Fluorescence intensity of 10,000 events was collected. Needle injury model Stable thrombi were induced in mesenteric veins of mice via mechanical disruption of the endothelium, using a microinjector needle tip (diameter 2–4 μm; Narishige PC-10 dual-stage glass micropipette puller, Tokyo, Japan). Needle injury was performed under direct vision (Nikon A1R microscope; or IX81 invert Olympus microscope, × 40 lens, Tokyo, Japan) using an Eppendorf InjectMan NI 2 micromanipulator to enable precise control of the needle (Eppendorf, Hamburg, Germany). The needle was passed into the vessel lumen, and then used to puncture the basal endothelium in a repetitive manner, such that endothelial injuries were performed in close proximity within a defined area (diameter ∼ 50 μm). Mechanical injury was either performed alone or in conjunction with local microinjection of platelet agonists (α-thrombin (100 Units ml −1 ), CRP or PAR4 peptide) as well as with catalytically inactive PPACK-α-thrombin, by positioning the needle ∼ 20–30 μm upstream from forming thrombi. Injections were performed using a programmable Femtojet injection system to ensure reproducibility (Eppendorf). Injections were programmed at 1,500 kpa for 1.5 s, resulting in delivery of ∼ 0.14 nl (ref. 69 ). Platelet thrombus formation and leukocyte migration were monitored via a combination of dissolved inorganic carbon (DIC) and epifluorescence microscopy (Olympus IX81 (Tokyo, Japan), and images captured using a QuantEM EMCCD camera (Tucson, AZ, USA)) or using confocal intravital microscopy (Nikon A1R). Where indicated, systemic injection of a PE-conjugated anti-Gr-1 Ab (100 μg kg −1 ) or DiOC6 (100 μg kg −1 )/DyLight 488/649 anti-GPIbβ antibody (100 μg kg −1 ) was performed to monitor leukocyte adhesion and thrombus formation, respectively. Mice were also systemically injected with FITC-PECAM-Ab (200 μg kg −1 ), Alexa 488/546-Annexin V (100 μg kg −1 ) or anti-fibrin-Alexa 488 Ab to identify endothelial cells, PS exposure and fibrin generation, respectively. In some experiments, mice were systemically administered hirudin (50 mg kg −1 ). Where platelet depletion was required, C57Bl/6J mice were administered an anti-GPIbα antibody (1 μg g −1 ; Emfret Analytics) via the inferior vena cava, and platelet count in peripheral circulation measured 10 min post administration to achieve a reduced platelet count of 0–1 × 10 6 μl −1 (KX-21 N Sysmex platelet analyser, Roche Diagnostics Australia Pty Ltd, Australia). For quantification of annexin V fluorescence following needle injury, single or repetitive injuries were induced in mice pre-administered with FITC-PECAM-Ab (200 μg kg −1 ) and Alexa 546-annexin V (100 μg kg −1 ). Confocal microscopy (Nikon A1R) was performed at the indicated post-injury time points. The total annexin V fluorescence (AU) on the injured endothelial cells was quantified using the NIS-Elements software (Nikon A1R) and specific annexin V binding determined by subtracting background annexin V fluorescence (measured before injury) from total annexin V fluorescence. Both thrombus surface area and volume were also quantified following needle injury. To quantify thrombus surface area, images of the thrombus near the base were captured using DIC (IX81 invert Olympus microscope, × 40). The ImageJ software (V1.45a NIH, USA) was then used to calculate the surface area by marqueeing the thrombus and calibrating the pixel size according to the magnification used. Thrombus surface area was quantified either at the indicated time post injury or between 2′30′ and 10′ post injury at 150′ intervals and expressed as an average. To quantify thrombus volume, thrombi were subjected to confocal sectioning (1 μm per section, Nikon AIR, × 40), the total number of fluorescent pixels from individual sections determined using the NIS-Elements software (Nikon AIR) and volumetric measurements obtained from summation of pixels from each section. Background fluorescence (in the adjacent area where there is no stable platelet adhesion) was subtracted from the total fluorescence. Captured confocal image stacks were also used to perform three-dimensional reconstruction of thrombi with associated leukocyte recruitment at sites of traumatic endothelial injury. This was achieved using in-built software tools available from both NIS-Elements software version 4.0 (Nikon A1R) and Imaris 7.6.4 software (Bitplane, Zurich, Switzerland). To quantify leukocyte migration post-needle injury, basal leukocyte migration was monitored at 5 s (12 frames per minute) intervals for up to 30 min, and analysed frame-by-frame using the ImageJ software (V1.45a NIH). Migrating leukocytes were defined as leukocytes that following contact with the thrombus underwent shape change to a polarized morphology and migrated a distance greater than or equal to one cell diameter towards the centre of the thrombus. Only leukocytes in the focal plane at the base of the thrombi were considered in this analysis. Analysis of leukocyte migration into the thrombus core was performed by demarcating the core (circular region, radius 25 μm) in the centre of the thrombus, reflecting the site of needle injury. Leukocyte migration velocity was calculated by tracking the migration of individual leukocytes at 50 s intervals for 10 min. Migration velocity was measured for each leukocyte using the ImageJ software (V1.45a NIH). Analysis of leukocyte recruitment by thrombi and endothelium The number of leukocytes stably adherent to the site of endothelial injury (with platelet depletion), or adherent to the margins or within the body of a thrombus, were quantified 20 min post injury. To account for differences in thrombus size, the results were normalized for thrombus surface area. In the case of platelet depletion, the number of leukocytes were normalized for the size of the initial area of injury (region of radius of 25 μm). Administration of rt-PA following needle injury Thrombi were induced in mesenteric veins by needle injury in combination with microinjection of α-thrombin in mice systemically injected with anti GPIbβ-DyLight 649 Ab, anti-Gr-1(RB6–8C5)-PE and anti-fibrin-Alexa 488 Ab. Leukocyte–thrombus interactions were monitored periodically using confocal microscopy (Nikon A1R) for up to 2.5 h. Recombinant tissue plasminogen activator (rt-PA—alteplase) was then administered at a dose of 30 mg kg −1 via a cannula inserted into the jugular vein (bolus 2 mg kg −1 and infusion of 28 mg kg −1 over 30 min). The dose of rt-PA was based on human dosing regimens and on the fact that the murine fibrinolytic system is ∼ 30-fold less sensitive to the effect of rt-PA than in humans [70] . Thrombolysis was confirmed by the loss of fibrin staining using confocal microscopy. Leukocyte migratory responses to the residual platelet mass were imaged using confocal microscopy following completion of the rt-PA infusion. In some experiments, α-thrombin or PPACK-α-thrombin was locally microinjected in the region of the residual platelet mass and the resultant thrombotic response monitored. The number of leukocytes migrating to the site of injury per unit area post rt-PA was quantified by averaging the ‘zone of exclusion’ of migration for pre-rt-PA thrombi, and then marqueeing an equivalent area within the residual platelet mass at the apparent site of injury post rt-PA and counting the number-polarized leukocytes within this zone. This result was normalized per unit area. Statistical analysis Statistical significance between multiple treatment groups was analysed using a one-way analysis of variance with Dunnett’s post-testing. Statistical significance between two treatment groups was analysed using an unpaired Student’s t -test with two-tailed P values (Prism software; GraphPAD Software for Science, San Diego, CA). Data are presented as means±s.e.m., where ‘ n ’ equals the number of independent experiments performed. How to cite this article: Kaplan, Z. S. et al . Thrombin-dependent intravascular leukocyte trafficking regulated by fibrin and the platelet receptors GPIb and PAR4. Nat. Commun. 6:7835 doi: 10.1038/ncomms8835 (2015).